Genome of the Chinese tree shrew Chinese tree shrews ( Tupaia belangeri chinensis ) possess many features valuable in animals used as experimental models in biomedical research. Currently, there are numerous attempts to employ tree shrews as models for a variety of human disorders: depression, myopia, hepatitis B and C virus infections, and hepatocellular carcinoma, to name a few. Here we present a publicly available annotated genome sequence for the Chinese tree shrew. Phylogenomic analysis of the tree shrew and other mammalians highly support its close affinity to primates. By characterizing key factors and signalling pathways in nervous and immune systems, we demonstrate that tree shrews possess both shared common and unique features, and provide a genetic basis for the use of this animal as a potential model for biomedical research. The tree shrew ( Tupaia belangeri ), currently placed in the order Scandentia, has a wide distribution in South Asia, Southeast Asia and Southwest China [1] . For several decades, owing to a variety of unique characteristics ideal in an experimental animal (for example, small adult body size, high brain-to-body mass ratio, short reproductive cycle and life span, low cost of maintenance, and most importantly, a claimed close affinity to primates) the tree shrew has been proposed as a viable animal model alternative to primates in biomedical research and drug safety testing [2] . Currently, there are many attempts to employ tree shrew to create animal models for studying hepatitis C virus (HCV) [3] and hepatitis B virus (HBV) infections [4] , myopia [5] , as well as social stress and depression [6] , [7] . Recent studies of aged tree shrew brain suggested that tree shrew is also a valid model for aging research [8] and learning behaviours [9] . Despite marked progress in using tree shrews as an animal model, tree shrews are studied only in a handful of laboratories worldwide, partially because there is no pure breed of this animal, limited access to this animal resource and lack of specific reagents. Moreover, a great number of obstacles to furthering these studies remain, especially the lack of a high-quality genome and an overall view of gene expression profiling that leave several key questions unanswered: (a) How closely related are tree shrews to primates; (b) do tree shrews share similarity of key signalling pathways to primates and be fully used as an adjunct to primates; and (c) what are the unique biological features of the tree shrew? The answers to these questions provide the information foundation needed to expedite current efforts in making the Chinese tree shrew a viable model animal, and to design and develop new animal models for human diseases, drug screening and safety testing. In this study, we presented a high-quality genome sequence and the annotation of Chinese tree shrew. Comparison of tree shrew and other genomes, including human, revealed a closer relationship between tree shrew and primates. We identified several genetic features shared between tree shrew and primates, as well as the unique genetic changes that corresponds to their unique biological features. The data provided here are a useful resource for researches using tree shrew as an animal model. Genome sequencing of the Chinese tree shrew To address the phylogenetic relationship and genetic divergence of tree shrew and human, and also facilitate the application of the Chinese tree shrew as an animal model for biomedical research, we generated a reference genome assembly from a male Chinese tree shrew ( Tupaia belangeri chinensis ) from Kunming, Yunnan, China. 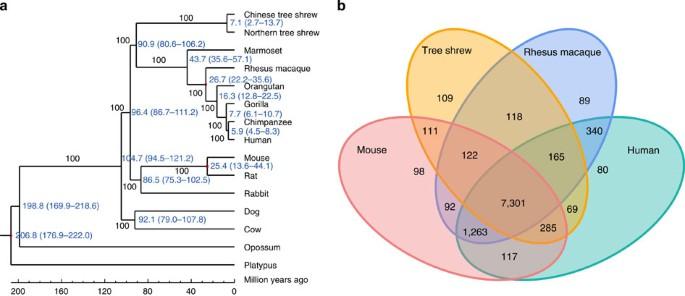Figure 1: Relationship of the Chinese tree shrew and related mammals. (a) Consensus phylogenetic tree of 15 (sub)species based on 2,117 single-copy genes. The topology was supported by all phylogenetic resources including full-coding sequences, first, second, third codon positions, and amino acids from the orthologous genes. Bootstrap values were calculated from 1,000 replicates and marked in each note. The divergence times for all notes were estimated using three notes with fossil records as calibration times and marked in each note with error range. (b) Venn diagram of Chinese tree shrew gene families with human, rhesus macaque and mouse. The assembly was generated with 79 × high-quality Illumina reads from 19 paired-end libraries with various insert sizes from 170 bp to 40 kb ( Supplementary Table S1 ), and has a contig N50 size of 22 kb and a scaffold N50 size of 3.7 Mb ( Table 1 ). The total assembled size of the genome is about 2.86 Gb, close to the 3.2 Gb genome size estimated from the K-mer calculation ( Supplementary Fig. S1 ). Repetitive elements comprise 35% of the tree shrew genome ( Supplementary Table S2 ). Unlike primate genomes, which are characterized by a large number of Alu/SINE elements, the tree shrew genome has a marginal proportion of this element but contains over a million copies of a tree shrew-specific transfer RNA-derived SINE (Tu-III) family, representing the dominated transposon that makes up 14% of the entire genome ( Supplementary Table S3 ). Table 1 Global statistics of the Chinese tree shrew genome. Full size table To aid the gene annotation of the tree shrew genome, we generated a high-depth transcriptome data from seven tissues including the brain, liver, heart, kidney, pancreas, ovary and testis collected from two Chinese tree shrews ( Supplementary Methods 1 ). The genome was then annotated with a method integrating the homologous prediction, ab initio prediction and transcription-based prediction methods ( Supplementary Methods 3.2 ). A non-redundant reference gene set included 22,063 protein-coding genes of which 17,511 genes show one-to-one orthology with other mammals, while the remaining genes display complicated orthologous relationships. We compared the major parameters of our genome assembly with the recently released tree shrew genome by Broad Institute ( http://www.ensembl.org/Tupaia_belangeri/Info/Index ; abbreviated as Broad version in the below text), and found that our assembly has great advantages than the Broad version ( Supplementary Table S4 ). First, the Broad version only provided very low coverage (2X) for the tree shrew genome, whereas we offered very high depth (~79X) coverage to guarantee a high accuracy for the genome at the single-base level. Second, our assembly is more complete than the Broad version. The contiguous non-gap sequences covered over 85% of our tree shrew genome, while the Broad version covered <67% of the genome. A more complete assembly allows us to perform a comprehensive analysis for the genomic features of this animal and to systemically compare with other species (see below). Third, our assembly provided over 20 times longer than the Broad version in the scaffold size. The assembly with longer scaffolds and contig scan allows us to produce a more complete individual gene model and a long gene synteny, which is very useful for cross-species comparisons. Finally, with the availability of our high-quality assembly, we generated a significantly improved annotation for the tree shrew genome, which contains 22,063 genes and is closer to the human gene number. In contrast, the gene annotation of the Broad version was based on the homological prediction and only includes 15,414 genes (most of them are partial genes). In addition, our gene models are supported by the high-depth transcriptome data. Over 95% of our gene models have complete open reading frames, while only <40% of gene models in the Broad version are complete. Overall, we provided a high-quality genome together with the well-annotated genes, which would be a very useful resource for the scientific community. Evolutionary status of the tree shrew The entire tree shrew genome sequence offers essential information needed to settle ongoing debates on the exact phylogenetic position of this species in Euarchontoglires [10] , [11] . Analyses of the mitochondrial genome showed that the tree shrew had a closer relationship to Lagomorpha than to Dermoptera or primates, [11] and molecular cytogenetic data supported a Scandentia–Dermoptera sister clade [10] . However, available evidence from multiple nuclear genes suggests a closer affinity of tree shrews and primates (including human) [12] , [13] . In a recent study by Hallström et al. [14] based on 3,000 genes for phylogenetic analysis, tree shrew was grouped with Glires (including Rodentia and Lagomorpha), suggesting a closer affinity of tree shrew with mouse or rabbits. However, this placement was insufficiently supported thus even unresolved. Genome sequencing of the Chinese tree shrew and comparison with 14 other species, including 6 primate species, on the basis of 2,117 single-copy genes showed that the tree shrew was first clustered with primate species with a high bootstrap support by all phylogenetic signals, including coding sequences with all codon positions and peptide sequences ( Fig. 1 and Supplementary Fig. S2 ). This result helped to clarify potential controversy regarding the phylogenetic position of tree shrew within eutherian mammals reconstructed on the basis of mitochondrial DNA genome [11] , genome-wide comparative chromosome map [10] and multilocus nuclear sequences [12] , [13] . It should be mentioned that we observed an unexpected deep split between our tree shrew and the one sequenced by the Broad Institute ( Supplementary Fig. S2 ). If this was not caused by the potential sequence quality owing to the low coverage of the Broad version, one would expect that the divergence of tree shrew from different geographic regions may be more complex albeit they were grouped as one species ( Tupaia balangeri ). Figure 1: Relationship of the Chinese tree shrew and related mammals. ( a ) Consensus phylogenetic tree of 15 (sub)species based on 2,117 single-copy genes. The topology was supported by all phylogenetic resources including full-coding sequences, first, second, third codon positions, and amino acids from the orthologous genes. Bootstrap values were calculated from 1,000 replicates and marked in each note. The divergence times for all notes were estimated using three notes with fossil records as calibration times and marked in each note with error range. ( b ) Venn diagram of Chinese tree shrew gene families with human, rhesus macaque and mouse. Full size image We estimated the divergence time among these 15 mammalian genomes ( Fig. 1 ). The tree shrew seems to have diverged from the clade encompassing the six primate species around 90.9 million years ago, whereas the rodent clade diverged from the primate clade relatively earlier, around 96.4 million years ago. The close affinity of tree shrews to non-human primates, as demonstrated by the clustering pattern in the phylogenetic tree and relatively smaller divergence time, directly settles controversies regarding the phylogenetic position of tree shrews within Euarchontoglires as well as supports rationale for using tree shrews as an adjunct and alternative to primates as animal models. Genetic relationship of tree shrews and humans The genetic basis of primate uniqueness and phenotypic distinctions is under intense scrutiny. The clustering of tree shrew and primates within the Euarchonta clade is consistent with the observation that the tree shrew genes have an overall higher similarity in proteins with humans than rodents ( Supplementary Fig. S3 ). The closer relationship between tree shrew and primates raises an interesting question: what primate genes emerged from the Euarchonta clade and are shared in the tree shrew genome? These genes may encode functional proteins that shape similar phenotypic characters between tree shrews and primates. From multiways gene synteny of humans, tree shrews and mice ( Supplementary Methods 4.5 ), we identified 28 genes previously considered primate specific present in the tree shrew genome that are likely to have originated in the Euarchonta clade ( Supplementary Table S5 ). One such example is the psoriasin protein, a potent chemotactic inflammatory protein that has an important role in the innate defence against bacteria on the surface of the body [15] , which has duplicated twice within the Euarchonta and formed three tandem duplicated gene clusters in both tree shrews and other primates, including humans. Another example is the NKG2D–ligand interaction, a powerful mechanism to activate natural killer cells and T cells that regulates immune recognition and responses during infection, cancer and autoimmunity [16] . The NKG2D ligands are induced in response to a variety of stress stimuli but these ligands belong to diverse families in humans and mice [17] . Tree shrews possess the same ligand families as humans, consisting of a major histocompatibility complex (MHC) class I-related chain ( MIC ) gene and the ULBP (UL16-binding protein) family ( Supplementary Fig. S4 ), and they have six members in the ULBP family, similar to humans [18] . This observation suggests that the tree shrews’ immune system may employ the same indicators as in humans to cue the elimination of infected, stressed and damaged cells. Unique genetic features of the tree shrew By comparing primate and rodent genomes, we identified several lineage-specific genetic changes that potentially contributed to the tree shrews’ adaptations. A total of 162 gene families underwent specific expansion in tree shrews ( Supplementary Methods ) with the immunoglobulin lambda variable gene family showing the most striking expansion, 67 copies in tree shrews but only 36 copies in the human genome ( Fig. 2a ). The immunoglobulins can block and promote elimination of the pathogen antigens, and accordingly, this expansion could provide an immediate selective advantage to tree shrews. To further investigate specific gene loss or pseudogenization in tree shrews, we compared the gene synteny of the tree shrew, human and mouse genomes. We identified a total of 11 (potential) gene loss and 144 pseudogenes in the tree shrew genome ( Supplementary Table S6 and Supplementary Data 1 ). Of particular interest, the prostate-specific transglutaminase 4 ( TGM4 ), which expresses as a seminal fluid protein, was lost in tree shrews. This protein participates in the formation or dissolution of seminal coagulum, a process that has an important role in sperm competition [19] . The absence of TGM4 may be consistent with the observed tree shrew mating system, for example, Tupaia tana species and a few other tupaiids are generally considered behavioural monogamy [1] , [20] , so competitive postmating is lacking in males of this species. Premature stop codon mutations or frame-shift mutations may also lead to functional loss of some important genes in the tree shrew, for example, the NADPH oxidase ( NOX1 ) gene, which has an important role in cellular defence against acidic stress [21] , was disrupted by a premature stop codon in tree shrews. The pseudogenization of this gene suggests that tree shrews may have reduced levels of reactive oxygen species in the arterial wall in conditions like hypertension, hypercholesterolaemia, diabetes and aging, as well as infection. 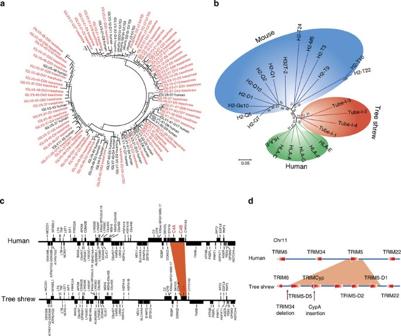Figure 2: Immune system in Chinese tree shrew and compared with human and mouse. (a) Specific expansion of the immunoglobulin lambda variable (IGLV) gene family in the tree shrew. Gene IDs in red are tree shrew genes. (b) Phylogenetic relationship of MHC-class I genes in human, tree shrew and mouse. (c) Highly conserved gene synteny of MHC-class III region between human and tree shrew. Black bar represents the gene in each species. (d) Trim gene cluster in tree shrew and human. Tree shrews have lostTRIM34while had multiple specific duplication ofTRIM5, one of which was inserted by CypA transposon, leading to a fused transcript Trim-Cyp. Figure 2: Immune system in Chinese tree shrew and compared with human and mouse. ( a ) Specific expansion of the immunoglobulin lambda variable ( IGLV ) gene family in the tree shrew. Gene IDs in red are tree shrew genes. ( b ) Phylogenetic relationship of MHC-class I genes in human, tree shrew and mouse. ( c ) Highly conserved gene synteny of MHC-class III region between human and tree shrew. Black bar represents the gene in each species. ( d ) Trim gene cluster in tree shrew and human. Tree shrews have lost TRIM34 while had multiple specific duplication of TRIM5 , one of which was inserted by CypA transposon, leading to a fused transcript Trim-Cyp. Full size image Nervous system of the tree shrew Tree shrews have a high brain-to-body mass ratio and a well-developed brain structure resembling primates [1] . Available evidence indicates that tree shrews could be used in depression research [6] . A dominant and subordinate relationship could be created between two male tree shrews in visual and olfactory contact, with the subordinate animal showing a remarkable alteration of physiological, brain functional and behavioural activities that are similar to those observed in depressed patients [6] . In humans, the polymorphism of the serotonin transporter promoter is reputedly associated with the stress disorder and depression susceptibility [22] . However, tree shrews lack this polymorphism region [23] , a finding confirmed by our genome sequencing, implying a potentially different regulation of this gene in stress reactions between tree shrews and humans. Excepting this difference, we detected all 23 known neurotransmitter transporters ( Supplementary Table S7 ) in the tree shrew genome that have known roles responsible for the corresponding features of depression [24] . Studies have demonstrated that antidepressants function in patients by suppressing the activity of neurotransmitter transporters [25] . In tree shrews, these transporters are highly conserved in amino-acid sequence with their human counterparts, with the exception of glycine transporter type 1 protein, which shows a relatively fast rate of evolution in the tree shrew lineage ( Supplementary Fig. S5 ). The existence of complete and conserved neurotransmitter transporters in tree shrews provides a genetic basis for making tree shrews an attractive model for experimental studies of psychosocial stress [6] and evaluation of pharmacological effect of antidepressant drugs. Similar to primates, tree shrews have an especially well-developed visual system, colour vision and eye structure [1] . A recent study reported that there is a close homology between cholinergic mechanisms in tree shrew and primate visual cortices [26] . Experiments on tree shrews suggest that the subordinate relationship caused by social stress is mediated by visual rather than olfactory cues [27] , coinciding with our finding that several olfactory genes have been pseudogenized and the relatively small number of observed olfactory receptors ( n =690) in tree shrews as compared with in rodents ( n =~1,000) ( Supplementary Methods ). The well-developed eye structure of tree shrews has also created substantial interest in using tree shrews as a model in ophthalmological studies, especially for myopia [5] . To provide a genetic basis for the tree shrews’ visual system, we systemically scanned the genes involved in visual system. The tree shrew genome encompasses the orthologues of almost all the 209 known visually related human genes, but lacks two cone photoreceptors, the middle wave-length sensitive proteins, which are specifically duplication genes in catarrhines and lead to the trichromacy in higher primates [28] . The absence of the middle wave-length sensitive proteins is consistent with the fact that tree shrews, similar to some lower primates, lack the green pigment and possess dichromats [29] . As most tree shrew species are diurnal and spend the entire night for sleep in their nests, they do not rely on dim-light visuals [29] . The evolutionary rate testing suggested that the rod photoreceptor rhodopsin, which is responsible for the night vision, had a faster evolutionary rate in the tree shrew lineage ( Supplementary Fig. S6 ), suggesting a looser evolutionary constraint of dim-light vision because of their adaptation to the diurnal life. Mutation p.F45L of rhodopsin can cause retinitis pigmentosa, an incurable night blindness disease in humans [30] . Interestingly, we detected a unique p.F45C substitution in tree shrew species ( Supplementary Fig. S7 ), which implies a potentially functional degeneration of this gene in tree shrews. This finding corroborates earlier observations of heavily cone-dominated retina structures with only a small proportion of rod photoreceptors in tree shrews [31] . In addition, we checked the presence of genes regulating the circadian photoreceptor, including both rod–cone photoreceptive systems and non-visual photoreceptive systems, in tree shrew and compared their sequence identity between tree shrew and human. We identified an overall high amino-acid sequence identity (except for enzyme acetylserotonin O -methyltransferase) for genes that are involved in photopigment, phototransduction or synthesis of melatonin, which acts as a circadian rhythm regulator [32] ( Supplementary Table S8 ). This pattern may explain why most tree shrews are day-active. Immune system of the tree shrew Hepatitis B is an inflammatory liver disease caused by HBV, which has infected about 2 billion people globally and with an annual death toll estimated at 600,000(ref. 33 ). Hepatitis C is caused by the HCV, another worldwide infectious disease [34] . Except for chimpanzees, there are many reports that tree shrew and its hepatocytes could be infected with human HBV [4] and HCV [3] . Hence, the property of genes involved in immunity response of viral infection demonstrated by tree shrews further contributes to their preferred choice as an attractive model for studying viral hepatitis and hepatocellular carcinoma [35] . Here, the available tree shrew genome data offer a distinct advantage to scan these immune genes involved in viral hepatitis. The MHC has a central role in immune responsiveness and susceptibility to various autoimmune and infection diseases. However, so far there is limited information for tree shrew MHC sequences [36] , [37] . Even though the fragment nature of MHC region and sequencing of the MHC in tree shrew are still incomplete, several points can be distilled from the genome data. First, the entire MHC region of tree shrews is conserved with that of humans, both in the organization of MHC and the gene syntenic order. Second, tree shrews bear at least four genes that belong to MHC class I genes, which are homologous to HLA class I gene and one MIC ( Supplementary Fig. S8 ). Phylogenetic tree analysis clusters tree shrew genes into a separated group diverging from human class I gene group, implying tree shrews have a unique MHC class I locus formed by paralogous amplification ( Fig. 2b ). Intriguingly, one class I gene in tree shrews is located in the HLA-A region and has well synteny with human locus. However, its functional orthologue with HLA class I gene requires further experimental inspection ( Supplementary Fig. S8 ). The MHC class II region of the tree shrew encompasses homologous of all human class II genes, including the classical class II gene HLA-DP , HLA-DQ and HLA-DR , as well as non-classical class II genes HLA-DM and HLA-DO ( Supplementary Fig. S9 and Supplementary Table S9 ). The class III region in tree shrews is the most conserved region with humans in gene syntentic alignment. However, in contrast with humans and mice that both obtained two copies of C4 by lineage-specific duplication [38] , tree shrews only have one C4 gene in this region ( Fig. 2c and Supplementary Fig. S10 ). We next investigated the property of gene interaction pathways involved in viral infection. Current studies suggest that a total of 163 human genes were reported to respond in HBV and HCV infection [39] , [40] . The counterparts of most of those genes are present in the tree shrew genome and shared a relatively high sequence identity with human ( Fig. 3 and Supplementary Data 2 ), with the exception of DDX58 . Tree shrews have lost DDX58 , which functions to trigger the transduction cascade involving in the signalling pathway mediated by the MAVS , resulting in the activation of NF-κB and is essential for the production of interferon in response to virus, including HCV [41] . The functional loss of DDX58 in tree shrews suggests that the interruption of immune response may serve as one potential reason causing the capable HCV infection in this animal. Interestingly, other subpathways involved in HCV infection show relatively lower cross-species genetic diversity than that of the MAVS–NF-κB signalling pathway ( Fig. 3 ), in which recurrent viral antagonism has led to a convergent evolution of escape from hepaciviral antagonism in primates [42] . Note that a recent study by Tong et al. [40] provided functional data that tree shrew CD81, SR-BI, claudin-1 and occludin support HCV infection. 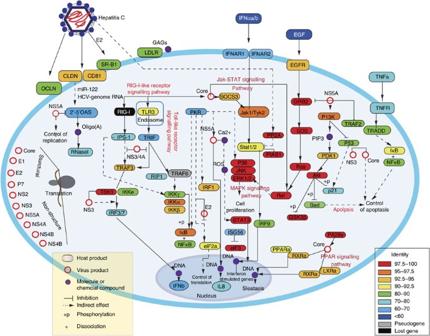Figure 3: Genetic divergence of genes involved in HCV infection pathway between human and Chinese tree shrew. Colours represent the degree of sequence identity at the amino-acid level. Figure 3: Genetic divergence of genes involved in HCV infection pathway between human and Chinese tree shrew. Colours represent the degree of sequence identity at the amino-acid level. Full size image Although HBV is classified as a double-stranded DNA virus, it behaves similarly to a retrovirus and replicates by reverse transcription of an RNA intermediate [43] . TRIM5 , one of the host restriction factors blocking retroviral replication [44] , is located in a gene cluster in human with three other closely related TRIM genes, including TRIM6 , TRIM34 and TRIM22 . Genes in this cluster have also been suggested to inhibit the activity of HBV [45] . In the tree shrew, this gene cluster displays a dynamic evolutionary episode ( Fig. 2d and Supplementary Fig. S11 ) as it has achieved five Trim5 copies with four encoding validated open reading frames by several lineage-specific tandem duplication events. Astonishingly, similar to some primates [46] , [47] , one of the TRIM5 copy has a CypA retrotranposition and form a TrimCyp chimera transcript, which was validated by reverse transcriptase PCR ( Supplementary Fig. S12 ). The appearance of TrimCyp independently in several primate species and tree shrews implies the potential importance of this fused transcript. The TRIM34 gene in the cluster, which also has function in retrovirus restriction [48] , however, has apparently been lost in tree shrews, though tree shrews may potentially have remedied the loss of TRIM34 with the expansion of TRIM5 . The current analysis for all related and essential genes involved in HBV and HCV infection ( Fig. 3 and Supplementary Data 2 ) provided helpful information for us to explain why this animal could be used to create animal model for viral infection. Although we did not provide independent infection experiments (either the animal or primary hepatocytes) to prove its susceptibility, the plenty of previous reports on HBV [4] and HCV [3] infection would certify tree shrews’ susceptibility to these viruses. Nonetheless, the findings for the absence of DDX58 gene and other unique gene features in tree shrew would account for the distinct immune response involved in viral hepatitis. Drug-targeted domain in tree shrews The cytochrome P450 (CYP) superfamily encodes the major enzymes involved in drug metabolism, activation and interaction [49] . In general, tree shrews have a more similar number of genes in CYP subfamilies with humans than mice do ( Supplementary Table S10 ). For example, mice have substantially expanded in CYP2 family with 46 members, while humans and tree shrews have fewer copy numbers. Finally, we sought to assess the genetic divergence of hepatitis drug-targeted genes between tree shrews and humans. A total of 42 genes are known targets for hepatitis drugs, such as halothane, theophylline and meperidine [50] , [51] . Only one gene, neuropeptide S receptor 1 ( NPSR1 ), has lost its targeted domain (7tm-1) of halothane in tree shrews owing to the frame-shift mutation ( Supplementary Fig. S13 ). All other druggable genetic components can be found in tree shrews and show high conservation in sequence with human orthologues ( Supplementary Table S11 ). The average diversity of the hepatitis drug-targeted domains between humans and tree shrews is about 5%. The conservation of the drug targets, together with the conserved signalling pathways in tree shrews and humans, would encourage the use of tree shrews as a substitution for human patients in pharmacokinetics evaluation of drug disposition, targets and side effects. Despite the fact that tree shrew has been proposed as a valid experimental animal to replace primates in biomedical research and drug safety testing [2] , there are limited usages of this animal in the field owing to many reasons. The publicly available annotated genome sequence of the Chinese tree shrew we generated offers an opportunity to decipher the genetic basis of the tree shrews’ suitability as an animal model for studying depression, myopia and viral infection [3] , [4] , [5] , [6] , [7] . Although we did not provide further experimental evidence to solidify the speculations deducted from the comparative genomics, the unique genetic features that we discerned from the genome of Chinese tree shrew has provided insightful information for us to understanding the biology of this animal. By comparing the overall genomic profile of tree shrews and other related mammalians, particularly those of the commonly used experimental animals like rats and mice, we showed that tree shrews had a relatively closer affinity to non-human primates, settling a long-running dispute regarding the phylogenetic position of tree shrew within the Euarchontoglires clade. We likewise characterized the key classes of molecules relevant to the tree shrew nervous and immune systems, demonstrating the genetic basis of this animal as a rising model for biomedical research. The availability of this new genomic data provides a valuable resource and tool for functional genomic and pharmacogenomic studies on tree shrews while also facilitating increasing use of the tree shrew as an animal model in broader fields. Source of samples A male Chinese tree shrew ( Tupaia belangeri chinensis ) from Yunnan, China, was used for DNA isolation and sequencing. RNA samples from the brain, liver, heart, kidney, pancreas and testis of another male Chinese tree shrew and from the ovary of one female individual were collected for transcriptome sequencing. All experiments on animals involved in this study have been approved by the Kunming Institute of Zoology Institutional Review Board. Genome sequencing and assembly DNA and RNA sequencing libraries were constructed using standard Illumina libraries prep protocols. Tree shrew genomes were assembled de novo by the de Bruijn graph-based assembler SOAPdenovo 1.05 (ref. 52 ). First, low-quality reads or those with potential sequencing errors were removed or corrected by K-mer frequency-based methods. SOAPdenovo1.05 constructed the de Bruijn graph by splitting the reads from short insert size libraries (170–800 bp) into 41-mers and then merging the 41-mers, after which the contigs (which exhibited unambiguous connections in de Bruijn graphs) were collected. All reads were aligned onto the contigs for scaffold building using the paired-end information. This paired-end information was subsequently used to link contigs into scaffolds, step-by-step, from short insert sizes to long insert sizes. Some intra-scaffold gaps were filled by local assembly using the reads in a read pair, where one end uniquely aligned to a contig while the other end was located within the gap. Genome annotation We employed RepeatMasker 3.3.0 (ref. 53 ) to identify and classify transposable elements by aligning the tree shrew genome sequences against a library of known repeats, Repbase ( http://www.girinst.org/repbase/ ), with default parameters. We used the same pipeline and parameters to re-run the repeat annotation in human, mouse, rat and dog genomes, which were downloaded from Ensembl (release 60). To predict genes in the tree shrew genome, we used both homology-based and de novo methods. For the homology-based prediction, human and mouse proteins were downloaded from Ensembl (release 60) and mapped onto the genome using TblastN 2.2.18. Then, homologous genome sequences were aligned against the matching proteins using GeneWise 2-2-0 (ref. 54 ) to define gene models. For de novo prediction, Augustus 2.5.5 (ref. 55 ) and Genscan 1.0(ref. 56 ) were employed to predict coding genes, using appropriate parameters. RNA-seq data were mapped to genome using Tophat 1.4.1(ref. 57 ), and transcriptome-based gene structures were obtained by cufflinks 1.3.0 ( http://cufflinks.cbcb.umd.edu/ ). Finally, homology-based, de novo -derived gene sets and transcript gene sets were merged to form a comprehensive and non-redundant reference gene set using GLEAN 2.0 ( http://sourceforge.net/projects/glean-gene/ ), removing all genes with sequences <50 amino acid as well as those that only had weak de novo support. Phylogenetic analysis We used TreeFam 7.0 ( http://www.treefam.org/ ) to define gene families among 15 mammalian genomes: human, chimpanzee, gorilla, orangutan, rhesus macaque, marmoset, Chinese tree shrew, northern tree shrew, rabbit, mouse, rat, dog, cow, opossum and platypus. We carried out the same pipeline and parameters used in our previously published study [58] . We obtained 18,823 gene families and 2,117 single-copy orthologues. The 2,117 single-copy gene families were used to reconstruct the phylogenetic tree. CDS sequences from each single-copy family were aligned by MUSCLE 3.7 ( http://www.ebi.ac.uk/Tools/msa/muscle/ ) with the guidance of aligned protein sequences and concatenated to one super gene for each species. Codons 1, 2, 3 and 1+2 sequences were extracted from CDS alignments and used as input for building trees, along with protein, CDS sequences. Then, RAxML 7.2.8 ( http://sco.h-its.org/exelixis/software.html ) was applied for these sequence sets to build phylogenetic trees under the GTR+gamma model for nucleotide sequences and BLOSUM62+gamma model for protein sequences. We used 1,000 rapid bootstrap replicates to assess the branch reliability in RAxML 7.2.8. Using MCMCtree in PAML 4.4 (ref. 59 ), we determined split times with approximate likelihood calculation. The alpha parameter for gamma rates at sites was set as that computed by baseml in the initial step. The MCMC process of PAML 4.4 MCMCtree was run to sample 1 million times with sample frequency set to 50, after a burn-in of 5 millions iterations. The ‘fine-tune’ parameters were set as ‘0.00356 0.02243 0.00633 0.12 0.43455’ to make acceptance proportions fall in interval (20 and 40%). For other parameters we used the defaults. We applied Tracer 1.4 ( http://beast.bio.ed.ac.uk/ ) to check convergence. Two independent runs were performed to confirm the convergence. Gene family expansion analysis was performed using CAFE 2.1 ( http://sites.bio.indiana.edu/~hahnlab/Software.html ). In CAFE, a random birth and death model was proposed to study gene gain and loss in gene families across a user-specified phylogenetic tree. A global parameter λ, which described both the gene birth ( λ ) and death ( μ =− λ ) rates across all branches in tree for all gene families was estimated using maximum likelihood. Then, the conditional P -value was calculated for each gene family, and families with conditional P -values less than threshold (0.05) were considered as having accelerated rate of expansion and contraction. Shared gene and loss gene identification To identify genes tree shrews and primates shared, we first elucidated the orthologous relationship among tree shrew, mouse and human proteins. The longest transcript from the Ensembl database (release 60) was chosen to represent each gene with alternative splicing variants. We then subjected all the proteins to BlastP analysis with the similarity cutoff threshold of e -value=1e −5 . With the human protein set as a reference, we found the best hit for each tree shrew protein in other species, with the criteria that >30% of the aligned sequence showed an identity above 30%. Reciprocal best-match pairs were defined as orthologues. Then gene order information was used to filter the false-positive orthologues caused by draft genome assembly and annotation. The orthologues not in gene synteny blocks were removed from further analysis. Previously identified primate-specific genes [60] were mapped on to the synteny map. Primate genes with tree shrew orthologues in the synteny map but which were absent in mice were considered candidate-shared genes between primates and tree shrews. We also performed the manual check for all candidate genes. From the synteny map, we also observed genes specifically missing in tree shrews that should have been lost in this species. To further confirm this finding, we manually checked and annotated the genes in the tree shrew genome, and filtered those located in gap regions. Pseudogene identification To detect homozygous pseudogenes in the tree shrew genome in silico , we first aligned all the human cDNA (Ensembl release-56) onto the tree shrew genomes using BLAT with parameters (–extendThroughN -fine). The best hit regions of each gene with 1-kb flanking sequence were cut down and re-aligned with their corresponding human orthologous protein sequence using GeneWise 2-2-0 (ref. 54 ) with parameters (-genesf -tfor -quiet), which could help define the detail exon–intron structure of each gene. All genes containing frame shifts or premature stop codons reported by GeneWise were considered candidate pseudogenes. We then carried out a series of filtering processes: (1) the reported frame shifts or premature stop codons were due to the flaw in algorithm of GeneWise that were filtered; (2) the candidate pseudogenes with obvious splicing errors near their frame shifts or premature stop codons were filtered; and (3) the candidate pseudogenes due to assembly error or heterozygosis were filtered. Finally, we compared all candidate pseudogenes with the alternative splicing forms in human. Accession codes: The Chinese tree shrew whole-genome shotgun project has been deposited at DDBJ/EMBL/GenBank under the accession number ALAR00000000. The version described in this paper is the first version, ALAR01000000. All short read data have been deposited into the Short Read Archive ( http://www.ncbi.nlm.nih.gov/sra ) under the accession number SRA055299 . Raw sequencing data of the transcriptome have been deposited in the Gene Expression Omnibus with the accession number GSE39150 . How to cite this article: Fan, Y. et al. Genome of the Chinese tree shrew. Nat. Commun. 4:1426 doi: 10.1038/ncomms2416 (2013).